Enantioselective Cu(I)-catalyzed borylative cyclization of enone-tethered cyclohexadienones and mechanistic insights 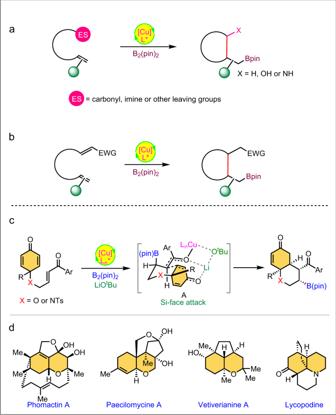Fig. 1: Previous and present approaches on Cu(I)-catalyzed borylative cyclization. aPrevious work: 1,2-Addition on various electrophilic sites (ES);bPresent work: 1,4-Addtion on α,β–unsaturated carbonyl compounds;cEnantioselective and diastereoselective desymmetrization of cyclohexadienone-tethered enones;dNatural products containing bicyclic pyran and hydroquinoline backbone. The catalytic asymmetric borylation of conjugated carbonyls followed by stereoselective intramolecular cascade cyclizations with in situ generated chiral enolates are extremely rare. Herein, we report the enantioselective Cu(I)-catalyzed β-borylation/Michael addition on prochiral enone-tethered 2,5-cyclohexadienones. This asymmetric desymmetrization strategy has a broad range of substrate scope to generate densely functionalized bicyclic enones bearing four contiguous stereocenters with excellent yield, enantioselectivity, and diastereoselectivity. One-pot borylation/cyclization/oxidation via the sequential addition of sodium perborate reagent affords the corresponding alcohols without affecting yield and enantioselectivity. The synthetic potential of this reaction is explored through gram-scale reactions and further chemoselective transformations on products. DFT calculations explain the requirement of the base in an equimolar ratio in the reaction, as it leads to the formation of a lithium-enolate complex to undergo C-C bond formation via a chair-like transition state, with a barrier that is 22.5 kcal/mol more favourable than that of the copper-enolate complex. Chiral Organoboranes are valuable synthetic intermediates in organic chemistry and the C–B linkage can be converted into C–C, C–O, and C–N bonds without racemization through stereospecific 1,2-migration [1] , [2] , [3] , [4] . Recently, copper has become a highly efficient and cost-effective catalyst for borylative addition with the diborane reagents on various functionalities [5] , [6] , [7] . Several reactions have been reported on tandem borylcupration of the carbonyls [8] , [9] , [10] , [11] , [12] , imines [13] , [14] , [15] , [16] , [17] , alkenes [18] , [19] , [20] , [21] , [22] , [23] , [24] , [25] , [26] , [27] , [28] , [29] , [30] , [31] , [32] , [33] , [34] , [35] , [36] , [37] , [38] , [39] , [40] , [41] , [42] , [43] , [44] , [45] , and alkynes [46] , [47] , [48] , [49] , [50] , followed by trapping with external electrophiles. However, copper-catalyzed borylative cyclization of alkene-tethered electrophiles has been rarely studied. Most of these intramolecular Cu-catalyzed tandem cyclization reactions investigated involve C–C bond formation via the alkylcuprate addition on carbonyls [51] , [52] , [53] , [54] , [55] , [56] , [57] , imines [58] , [59] , [60] , and various electrophilic carbon center bearing leaving groups (Fig. 1a ) [61] , [62] , [63] , [64] , [65] , [66] , [67] . In addition, the copper-catalyzed borylative reaction is a more convenient approach for ligand-assisted enantiocontrol cyclization [51] , [52] , [53] , [54] , [55] , [56] , [57] , [58] , [59] , [60] , [61] , [62] , [63] , [64] , [65] , [66] , [67] . Still, enantioselective Cu-catalyzed conjugate addition of nucleophilic boron followed by enolate trapping via aldol-addition or nucleophilic substitution is limited to not more than three reports. Lam et al. [51] , and Fernández et al. [57] reported the elegant enantioselective conjugate borylation/intra-molecular 1,2-addition strategy for the construction of densely functionalized fused carbocycles. Very recently, the research group of Lautens disclosed copper-catalyzed enantioselective conjugate borylation/Mannich cyclization to access enantioenriched tetrahydroquinolines [58] . However, to the best of our knowledge, Cu-catalyzed tandem conjugate borylation/intramolecular Michael addition has not yet been studied. Herein, we report the Cu-catalyzed asymmetric borylative annulation of C 2 -symmetric enone-tethered cyclohexadienones (bis-enones) (Fig. 1b ). Fig. 1: Previous and present approaches on Cu(I)-catalyzed borylative cyclization. a Previous work: 1,2-Addition on various electrophilic sites (ES); b Present work: 1,4-Addtion on α,β–unsaturated carbonyl compounds; c Enantioselective and diastereoselective desymmetrization of cyclohexadienone-tethered enones; d Natural products containing bicyclic pyran and hydroquinoline backbone. Full size image Over the last decade, enantioselective desymmetrization of prochiral cyclohexadienones has emerged as the most powerful and convenient strategy for the rapid construction of highly functionalized bicyclic frameworks in a single operation [68] , [69] , [70] , [71] , [72] , [73] , [74] , [75] , [76] , [77] , [78] , [79] , [80] , [81] , [82] , [83] , [84] , [85] . We have also been developing enantioselective Rh-catalyzed cyclizations of alkyne-tethered cyclohexadienones [86] , [87] , [88] , [89] , [90] , [91] , [92] , [93] . However, there are only two communications on the asymmetric borylative cyclization on alkene- or alkyne-tethered cyclohexadienones to give chiral cis-hydrobenzofurans. In 2013, Lin and co-workers reported Cu-catalyzed enantioselective borylative cyclization of O-tethered cyclohexadienone-containing 1,6-enynes using bis(pinacolato)diboron (B 2 pin 2 ) as a borylation reagent [77] . Here, the key regioselective borylcupration was achieved through O-directing coordination of the Cu-catalyst with propargyl ether. Subsequently, they further developed Rh(III)-catalyzed borylative annulation of alkene-tethered cyclohexadienones with excellent enantioselectivity [94] . Recently, our group [89] and Lu et al. [75] , investigated the reactivity of enone-tethered cyclohexadienone using the Friedel–Crafts alkylation of indole and the Rauhut–Currier reaction, respectively. In this work, we explore the copper-catalyzed β-borylative cascade annulation of enone-tethered cyclohexadienones to access chiral bicyclic pyran and hydroquinoline scaffolds via enantioselective desymmetrization (Fig. 1c ). The prevalence of these key structural motifs in a wide range of bioactive natural products highlights the emerging importance of borylative cyclization (Fig. 1d ). The reaction proceeds through conjugate borylation of enone and subsequent intramolecular Si-face attack of chiral enolate on the cyclohexadienone ring via a six-membered chair-like transition state, as depicted in intermediate A , fixing the stereochemistry at the four new contiguous stereocenters. However, the major challenge of this reaction is the chemoselective 1,4-addition of nucleophilic boron on three different enone-functionalities within the starting substrate and diastereoselective C–C bond formation. Optimization studies Our studies commenced with optimization of the racemic reaction conditions using cyclohexadienone-tethered enone 1a as a model substrate and (rac)-BINAP L1 (5 mol%) as ligand in THF (0.1 M) solvent at 0 °C (Fig. 2 , entries 1–8). The reaction with B 2 (pin) 2 (1.1 equiv) in the presence of Cu(CH 3 CN) 4 PF 6 (2.5 mol%) and NaO t Bu (0.1 equiv) afforded a trace amount of the desired product 2a along with significant quantity of uncyclized borylation product 3a (entry 1). When the base loading was increased (2 equiv), the required bicyclic product 2a was obtained exclusively in 78% yield (entry 4). Later, several bases such as K t OBu, K 2 CO 3 , Cs 2 CO 3 , and Li t OBu were subjected to borylative cyclization, and the yield of 2a was significantly improved, especially with Li t OBu (entry 8). Next, various representative chiral bisphosphine ligands ( L2 – L8 ) were examined in the presence Li t OBu as a base (entries 9–18). To our delight, (S)-SEGPHOS controlled the enantioselectivity remarkably well, affording the bicyclic product 2a in excellent yield (92%) with a high enantiomeric ratio at 0 °C (entry 10). Further optimization revealed that decreasing the reaction temperature (−78 °C) improved the enantiomeric ratio drastically (96:4) without significant loss of reaction yield (entry 13). However, the effect of other ligands ( L3 – L8 ) was also evaluated under the optimized conditions: either low yields or low enantioselectivity was observed in all the cases (entries 14-18). Overall, the desymmetrization of bis-enone 1a took place smoothly in the presence of ( S )-SEGPHOS at −78 °C, affording the desired bicyclic product 2a in 92% yield with 96:4 er (entry 13). Fig. 2: Evaluation of enantioselective Cu(I)-catalyzed borylative cyclization. Optimization of reaction conditions with various ligands and bases. Full size image Substrates scope Later, we investigated the versatility of asymmetric borylative cyclization of various enone-tethered cyclohexadienones 1 under optimized reaction conditions (Fig. 3 ). A variety of alkyl groups at the substrate′s prochiral quaternary center gave the corresponding bicyclic enones 2a – 2e in 89–92% yields with >92:08 er and excellent diastereoselectivities (>20:1). Moreover, methyl- and silyl-ether containing alkyl groups were also well tolerated ( 2f and 2g ). The reactions of benzyl, isopropyl, and cyclohexyl substituents at the enone quaternary center gave products 2h – 2j in 84–89% yield with higher enantiomeric ratios. In the case of the sec-butyl substituent, the product 2k was obtained as a 1:1 ratio of inseparable diastereomers relative to the stereocenter on the secondary butyl group. However, the sterically hindered tert-butyl group gave a lower enantiomeric ratio (entry 2l ). The reaction of substrates with aryl rings at the prochiral center was highly enantioselective with excellent yields ( 2m and 2n ). Interestingly, substrates with alkoxy substituents were also well tolerated in this reaction but with slightly lowered enantioselectivity (entries 2o – 2q ). Later, the reactivity of substituents on the arylketone backbone was also evaluated. All para-substituted arylketones gave good to excellent yields, regardless of their electronic properties (entries 2r – 2x ). However, it is interesting to note that the strong nature of electron-rich or electron-poor groups (OMe or CN) affected the enantiomeric ratio only slightly. Unfortunately, α,β-unsaturated olefins substituted with ester, aldehyde, and methyl ketone functionalities failed to give the desired products 2y , 2z , and 2za , due to lack of sufficient electrophilicity of the enone and most of the starting material was decomposed. The borylation on the substrate with the methyl group at the α-position of the cyclohexadienone ring afforded the required product 2zb in 24% yield, along with a significant quantity of the uncyclized product 2zb′ due to the steric effect. The reaction was also compatible with the bis(neopentyl glycolato)diboron reagent, giving the corresponding product 2zc in good yield with 86:14 er. However, other diboron reagents such as tetrahydroxydiboron and bis(catecholato)diboron failed to give the desired products. Interestingly, the optimized reaction conditions were also compatible with the NTs-linked substrate to provide the desired product 2zd in excellent enantioselectivity, albeit with a low yield. We also found that the yield of the borylated product significantly drops and that it has moderate stability during purification via silica gel column chromatography. The relative syn-syn-syn-syn configuration and absolute stereochemistry of the bicyclic enone 2n were unambiguously determined through X-ray crystallography, and the stereochemistry of all products was assumed by analogy (Fig. 3 ). Fig. 3: Substrate scope for O -tethered cyclohexadienones. Reaction conditions: 1 (0.3 mmol), B 2 (pin) 2 (84 mg, 0.33 mmol), Cu(CH 3 CN) 4 PF 6 (2.8 mg, 2.5 mol%), ( S )-SEGPHOS (9 mg, 5.0 mol%), t BuOLi (53 µL, 0.6 mmol, 1.0 M THF solution) in THF solvent (3 mL, 0.1 M). Isolated yields after column chromatography. Enantiomeric ratio (er) was determined by HPLC analysis using a chiral stationary phase. For most of the examples, >20:1 dr was observed from 1 H NMR analysis of isolated product 2 (see ESI). Full size image Next, we investigated the reactivity of the C-tethered enone 4 under standard reaction conditions (Fig. 4a ). The borylative cyclization still proceeded to give the annulation product 5 as a 2:3 ratio of inseparable diastereomers in 47% yield with 91:9 er and 85:15 er, respectively. In addition, the β-borylation/aromatization product 6 was also observed in 35% yield with 80:20 er. The formation of diastereomers and aromatization probably occurred due to the absence of the Thorpe-Ingold effect during C–C bond formation. 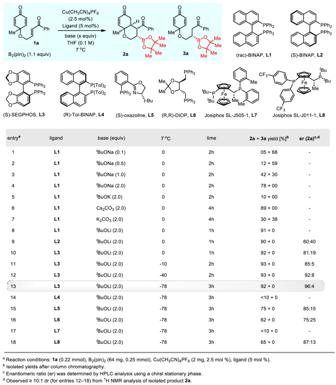Fig. 2: Evaluation of enantioselective Cu(I)-catalyzed borylative cyclization. Optimization of reaction conditions with various ligands and bases. Interestingly, in the case of the racemic cyclohexadienone 7 as a substrate, the annulation product 8 was observed in 41% yield with 96:4 er from only 50% of (R)- 7 isomer via parallel kinetic resolution (Fig. 4b ). However, we were unable to isolate product 9 from the (S)-isomer, and decomposition was observed. Fig. 4: Borylative cyclization. a Borylative cyclization of C-tethered substrate 4 ; b parallel kinetic resolution of racemic dienone 7 . Full size image Encouraged by the results discussed above, we sought to evaluate the one-pot sequential borylative cyclization/oxidation (Fig. 5 ). The Cu-catalyzed borylation of enone 1 under standard reaction conditions followed by the sequential addition of the sodium perborate oxidizing agent in the same flask afforded the β-alcohol product 10 via the β-borylation intermediate 2 . All reactions proceed with complete retention of stereochemistry, from the C–B bond to the C–O bond in a highly enantioselective fashion, and afforded the corresponding products 10a – 10l in similar yields and enantiomeric ratios, as compared to Fig. 3 . The relative stereochemistry was established by single-crystal X-ray analysis of compound 10a . It is worth mentioning that the phenyl-tethered enone was well tolerated in the annulation reaction to afford the corresponding product 10m in 61% yield. The sequential borylation/oxidation of the substrate with methyl groups at the α-position of the cyclohexadienone ring afforded the annulation product 10n in 44% yield in a 1:7:7.5:12 ratio of inseparable diastereomers. Regardless of the electronic properties of all substrates, we did not observe a propensity towards β-hydroxy elimination during the course of the reaction. In addition, one-pot sequential borylative cyclization/oxidation of N-tethered substrates gave the corresponding products 10o – 10r in 27–38% yield with excellent enantioselectivity and moderate to good diastereoselectivity. The low yield and high er is presumably a consequence of the steric effect from the NTs group. Fig. 5: One-pot sequential borylative cyclization/oxidation. Reaction conditions: Same as in Fig. 3 and then NaBO 3 .H 2 O (150 mg, 1.5 mmol, 5 equiv) was added in the same reaction flask and stirred at rt for 3 h. Isolated yields after column chromatography. Enantiomeric ratio (er) was determined by HPLC analysis using a chiral stationary phase. 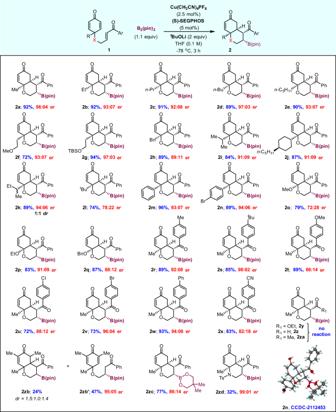Fig. 3: Substrate scope forO-tethered cyclohexadienones. Reaction conditions:1(0.3 mmol), B2(pin)2(84 mg, 0.33 mmol), Cu(CH3CN)4PF6(2.8 mg, 2.5 mol%), (S)-SEGPHOS (9 mg, 5.0 mol%),tBuOLi (53 µL, 0.6 mmol, 1.0 M THF solution) in THF solvent (3 mL, 0.1 M). Isolated yields after column chromatography. Enantiomeric ratio (er) was determined by HPLC analysis using a chiral stationary phase. For most of the examples, >20:1 dr was observed from1H NMR analysis of isolated product2(see ESI). For all examples, >30:1 dr was observed from 1 H NMR analysis of isolated product 10 . Full size image Next, we investigated the sequential borylative cyclization/oxidation in the absence of base under standard conditions (Fig. 6 ). Interestingly, the transformation on 1a led us to find fused dioxane 11a via conjugate borylation/oxidation/oxa-Michael addition instead of the C-Michael adduct 10a in 73% yield with moderate enantioselectivity [95] . It is evident that the absence of base (LiO t Bu) has a significant effect on the enantioselectivity. The relative stereochemistry was also established by single-crystal X-ray analysis of compound 11a . Other examples, including the enone bearing electron-deactivating 4-bromo phenyl ring and phenyl-tethered enone, also provided oxa-Michael products with moderate er (entries 11b , 11c , and 11e ), along with a trace quantity (>10%) of C-Michael products. In contrast, the strong electron-withdrawing nitro group failed to give the corresponding product 11d and the starting material was observed to decompose. Interestingly, the C-Michael addition was seen to be faster in the case of enones having the electron-rich aryl ring, affording the corresponding products 10g , 10h , and 10k , albeit with a moderate enantiomeric ratio. The substrate containing the aryl group at the quaternary carbon center also gave the C -Michael adduct 10f in 52% yield with 76:24 er. It is very interesting to note that cyclization is more favorable than β-hydroxy elimination under these reaction conditions. Fig. 6: One-pot sequential borylative cyclization/oxidation without a base. Reaction conditions: Same as in Fig. 3 , without t BuOLi base and then NaBO 3 .H 2 O (150 mg, 1.5 mmol, 5 equiv) was added in the same reaction flask and stirred at rt for 3 h. Isolated yields after column chromatography. Enantiomeric ratio (er) was determined by HPLC analysis using a chiral stationary phase. 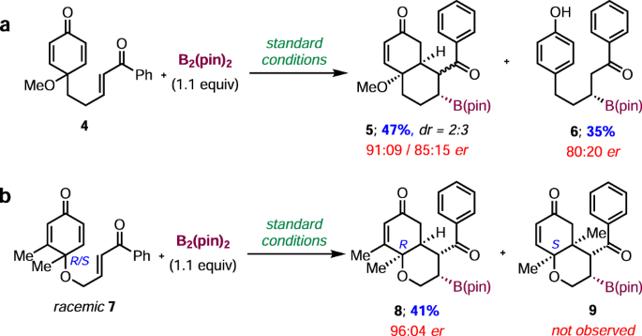Fig. 4: Borylative cyclization. aBorylative cyclization of C-tethered substrate4;bparallel kinetic resolution of racemic dienone7. For all examples, exclusive diastereoselectivity was observed from 1 H NMR analysis of isolated products 10 and 11 . Full size image DFT and mechanistic studies To understand the role of the base in the C–C bond formation and to find the factors leading to the diastereoselectivity, density functional theory (DFT) calculations were carried out using the Gaussian 09 program by employing the M06/SDD-6-311 + G(d,p)//B3LYP/SDD-6-31G(d) level of theory (details in the ESI). Before investigating the mechanistic pathway, we estimated the free energy required for the formation of the active catalyst [(S)-SEGPHOS-Cu-Bpin]. This process, which involves the addition of B 2 (Pin) 2 to the precatalyst, leading to the formation of the boryl copper complex, was found to be exergonic (Δ G = −18.8 kcal/mol). A distorted trigonal planar geometry around the coordination sphere of copper was observed for the active boryl copper complex (Fig. 7 ). Fig. 7: The optimized model of the boryl copper-complex [(S)-SEGPHOS-Cu-Bpin]. Hydrogen atoms have been removed for the purpose of clarity. Full size image The mechanism determined by DFT is as follows: once the catalyst is activated, the substrate 1a binds at the copper center to form a π-complex Int-1 , which is 2.3 kcal/mol (Δ G ) more favorable compared to the reactants taken separately (Fig. 8 ). The π-complex then undergoes 1,4-addition along the Cu-B bond to form Int-2 , which is highly thermodynamically favorable ( Int-2 , Δ G = −29.5 kcal/mol), which immediately converts to Int-3 (Δ G = −4.9 kcal/mol), allowing the B–O interaction. This step also explains the ambiguity regarding the axial position of Bpin. 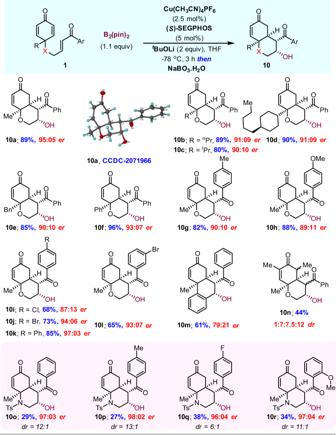Fig. 5: One-pot sequential borylative cyclization/oxidation. Reaction conditions: Same as in Fig.3and then NaBO3.H2O (150 mg, 1.5 mmol, 5 equiv) was added in the same reaction flask and stirred at rt for 3 h. Isolated yields after column chromatography. Enantiomeric ratio (er) was determined by HPLC analysis using a chiral stationary phase. For all examples, >30:1 dr was observed from1H NMR analysis of isolated product10. Bpin forms the B–O bond by overcoming a kinetic barrier of only +5.6 kcal/mol (Supplementary Fig. 4) . This stabilizes the system by 4.9 kcal/mol, as mentioned earlier. Hence, Bpin prefers the axial position, as upon moving to the equatorial position, it will lose out on the stabilizing B–O interactions. Following the formation of Int-3 , a rotation along the C–C(Ph)CO bond allows the carbon-bound copper to bind with oxygen, leading to the formation of Int-4 . This was found to be almost similar in energy w.r.t to the Int-3 , i.e, +0.5 kcal/mol (Δ G ). The crucial role of the extra LiO t Bu was then investigated and it was found that its absence leads to a pathway where the C–C bond formation for cyclization via a copper-enolate complex ( Int-5′ ) requires the overcoming of a kinetic barrier (TS-CC′) of +28.4 kcal/mol (w.r.t. to the most stable intermediate Int-2 ), which cannot be achieved at the reaction temperature (−78 °C), hence rendering the path unfavorable. However, the presence of that extra LiO t Bu allows Int-4 to form a more favorable (ΔΔ G = −25.0 kcal/mol, w.r.t Int-5′ ) lithium-enolate complex Int-5 . 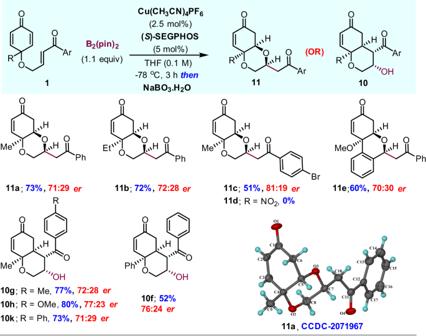Fig. 6: One-pot sequential borylative cyclization/oxidation without a base. Reaction conditions: Same as in Fig.3, withouttBuOLi base and then NaBO3.H2O (150 mg, 1.5 mmol, 5 equiv) was added in the same reaction flask and stirred at rt for 3 h. Isolated yields after column chromatography. Enantiomeric ratio (er) was determined by HPLC analysis using a chiral stationary phase. For all examples, exclusive diastereoselectivity was observed from1H NMR analysis of isolated products10and11. This leads to a transition state where lithium is in a position to interact with all the three oxygen atoms (two from the substrate and one from the O t Bu; see Supplementary Fig. 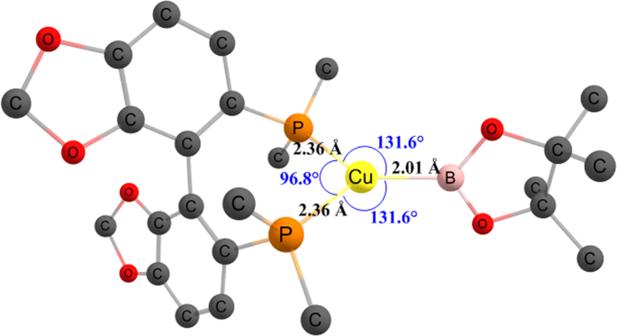Fig. 7: The optimized model of the boryl copper-complex [(S)-SEGPHOS-Cu-Bpin]. Hydrogen atoms have been removed for the purpose of clarity. 6 ), which plays a significant role in lowering the kinetic barrier (TS) needed for the cyclization (C–C bond formation) to +5.9 kcal/mol. This barrier is low enough that it can be overcome even at a low reaction temperature. This pathway also leads to the highly exergonic intermediate Int-6 , where the copper complex is already in a position to be released as the pre-catalyst (L n Cu–O t Bu). 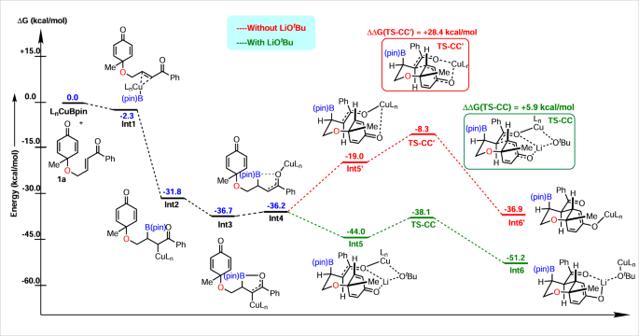Fig. 8: Computed free energy pathway. All the values are in kcal/mol with respect to the separate reactants LnCu-Bpin and substrate1a. Figure 8 depicts the complete energy pathway as discussed and all the relevant transition states are shown in Supplementary Figs. 4 and 5 in the ESI. Fig. 8: Computed free energy pathway. All the values are in kcal/mol with respect to the separate reactants L n Cu-Bpin and substrate 1a . Full size image Based on the above experimental results and DFT calculations, we propose the catalytic cycle shown in Fig. 9 . The reaction starts with the formation of ligated copper-complex L n Cu-O t Bu, resulting from Cu(CH 3 CN) 4 PF 6 , t BuOLi, and SEGPHOS. The transmetalation of L n Cu-O t Bu with B 2 pin 2 forms the active species L n Cu-B(pin), which undergoes borocupration of enone 1a via 1,4-addition to produce the alkyl-copper(I) complex A . 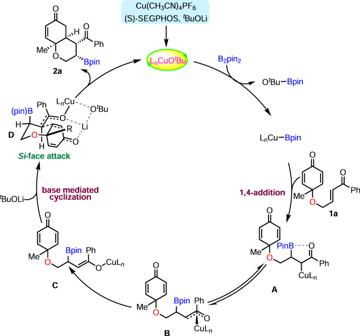Fig. 9: Plausible mechanism. The more favorable lithium-enolate undergoes a Si-face attack on the cyclohexadienone ring via a six-membered chair-like transition state to fix the contiguous stereocenters. 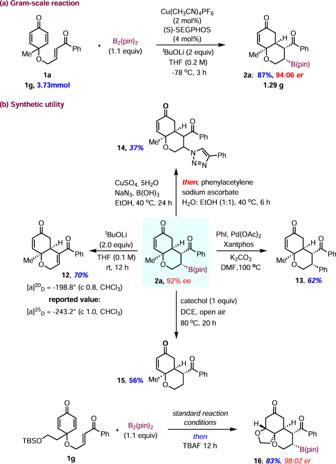Fig. 10: Gram-scale reaction and synthetic utility. aBorylative cyclization of substrate1ain 3.73 mmol (1.0 g) scale;bfurther transformations on product2a; one-pot borylation/oxa-Michael addition of substrate1g. Subsequently, Intermediate A equilibrates with the oxa-π-allylcopper species B to produce the reactive copper-enolate C , which does not undergo C–C bond formation due to the high kinetic barrier (ΔΔ G# = + 28.4 kcal/mol). As a result, transmetalation of intermediate C with excess LiO t Bu provides the lithium-enolate D and regenerates the active catalyst L n Cu-O t Bu. The more favorable (ΔΔ G = −25.0 kcal/mol) lithium-enolate D further undergoes a Si-face attack on the cyclohexadienone ring via a six-membered chair-like transition state to fix the contiguous stereocenters, as depicted in product 2a . Fig. 9: Plausible mechanism. The more favorable lithium-enolate undergoes a Si-face attack on the cyclohexadienone ring via a six-membered chair-like transition state to fix the contiguous stereocenters. Full size image Synthetic utility In order to demonstrate the synthetic utility, we carried out a gram-scale reaction on 1a with a slightly reduced catalyst loading under standard conditions (Fig. 10a ). A similar range of enantioselectivity of 2a was observed with 87% yield and it was further subjected to base mediated elimination to afford the known bicyclic enone 12 [75] in 70% yield (Fig. 10b ). The absolute stereochemistry was again confirmed by the optical rotation of enone 12 , which is consistent with the X-ray crystallographic analysis of compound 2n . In addition, the Pd-catalyzed Suzuki–Miyaura cross-coupling reaction of boronate 3a with phenyl iodide allowed the installation of the aryl ring at the β-carbon to give the corresponding product 13 in 62% yield [96] , [97] , [98] . A copper-catalyzed one-pot in situ azidation/[3 + 2]-cycloaddition of boronate 2a with NaN 3 and phenylacetylene provided 1,2,3-triazole 14 in moderate yield [99] . To further highlight the importance of this method, organoborane 2a was converted to the corresponding alkane 15 via a mild radical-mediated C–B cleavage, with simple catechol in the presence of open air [100] . One-pot sequential borylative cyclization of silyl-ether 1g under standard conditions, followed by addition of TBAF in the same reaction flask afforded the tricyclic product 16 in 83% yield and 98:2 er with exclusive diastereoselectivity via the desilylation/oxa-Michael reaction. Fig. 10: Gram-scale reaction and synthetic utility. a Borylative cyclization of substrate 1a in 3.73 mmol (1.0 g) scale; b further transformations on product 2a ; one-pot borylation/ oxa -Michael addition of substrate 1g . Full size image In summary, we have developed the enantioselective Cu(I)-catalyzed β-borylation/Michael addition of prochiral enone-tethered 2,5-cyclohexadienones. The reaction proceeds via 1,4-borocupration at the enone followed by a Si-face attack of chiral enolate on the cyclohexadienone ring via a chair-like transition state. DFT calculations explain the requirement of the excess base, leading to the formation of the more favorable chiral lithium-enolate, which undergoes C–C bond formation in the key desymmetrization step. One-pot sequential borylation/cyclization/oxidation afforded the corresponding alcohols without affecting the yield and enantioselectivity. This asymmetric desymmetrization strategy has broad substrate scope, generates highly functionalized bicyclic enones bearing four contiguous stereocenters with excellent yield, enantioselectivity, and diastereoselectivity offers new prospects in the rapid synthesis of highly functionalized structural motifs. The synthetic utility of this reaction has been demonstrated with a gram scale reaction and further chemoselective transformations on the product 2a . Further studies on the related asymmetric cyclizations of prochiral cyclohexadienones are underway in our laboratory. General procedure for the borylative cyclization reaction A solution of Cu(CH 3 CN) 4 PF 6 (2.8 mg, 2.5 mol%), ( S )-SEGPHOS (9 mg, 5 mol%), B 2 (pin) 2 (84 mg, 0.33 mmol), and t -BuOLi (53 µl, 0.6 mmol, 1 M in THF) in dry THF (2.0 mL) was stirred at room temperature for 15 min and then maintained at −78 °C. A solution of enone 1 (0.3 mmol) in dry THF (1.0 mL) was added via syringe and the resulting mixture was stirred at −78 °C for 3 h. The reaction mixture was quenched with saturated NH 4 Cl (10 mL) solution and extracted with EtOAc (3 × 15 mL) and dried over anhydrous Na 2 SO 4 , filtered, and concentrated in vacuo. The resultant crude product 2 was purified by column chromatography (hexanes/EtOAc). General procedure for the one-pot sequential borylative cyclization/oxidation reaction A solution of Cu(CH 3 CN) 4 PF 6 (2.8 mg, 2.5 mol%), ( S )-SEGPHOS (9 mg, 5 mol%), B 2 (pin) 2 (84 mg, 0.33 mmol), and t BuOLi (0.53 µl, 0.6 mmol, 1 M in THF) in dry THF (2.0 mL) was stirred at room temperature for 15 min and then maintained at −78 °C. A solution of enone 1 (0.3 mmol) in dry THF (1.0 mL) was added via syringe and the resulting mixture was stirred at −78 °C for 3 h then NaBO 3 ·H 2 O (150 mg, 1.5 mmol) in H 2 O (2 mL) was added in one portion and the resulting mixture was stirred vigorously at room temperature for 3 h under open air. The reaction mixture was quenched with saturated NH 4 Cl solution (10 mL) and extracted with EtOAc (3 × 15 mL) and dried over anhydrous Na 2 SO 4 , filtered, and concentrated in vacuo. The resultant crude product 10 was purified by column chromatography (hexanes/EtOAc).